The pyrido[b]indole MDM2 inhibitor SP-141 exerts potent therapeutic effects in breast cancer models A requirement for Mouse Double Minute 2 (MDM2) oncogene activation has been suggested to be associated with cancer progression and metastasis, including breast cancer. To date, most MDM2 inhibitors have been designed to block the MDM2–p53-binding interphase, and have low or no efficacy against advanced breast cancer with mutant or deficient p53. Here we use a high-throughput screening and computer-aided, structure-based rational drug design, and identify a lead compound, SP-141, which can directly bind to MDM2, inhibit MDM2 expression and induce its autoubiquitination and proteasomal degradation. SP-141 has strong in vitro and in vivo antibreast cancer activity, with no apparent host toxicity. While further investigation is needed, our data indicate that SP-141 is a novel targeted therapeutic agent that may especially benefit patients with advanced disease. Breast cancer has become the most frequently diagnosed cancer among women in the United States and is the second leading cause of cancer-related death in women [1] , [2] . In addition to advanced age, excessive exposure to oestrogens and a deficiency in the maintenance of genomic integrity have been considered as the two major reasons for a high breast cancer risk [3] . Despite an early diagnosis and new treatment options, such as less drastic surgery, novel chemotherapeutic agents and radiotherapy regimens, which have contributed to improved survival and quality of life for breast cancer patients, the mortality rate is still high for patients with advanced breast cancer [4] , [5] . In addition, molecular-targeted therapies, such as selective oestrogen receptor modulators, aromatase inhibitors and human epidermal growth factor receptor 2 antagonists have been successfully developed and helped to increase survival but have limitations because of intrinsic alternations of multiple molecules or genes at the genetic and epigenetic levels [6] , [7] . In particular, triple-negative breast cancers (TNBCs, lacking the expression of the oestrogen receptor (ER), progesterone receptor (PR) and human epidermal growth factor receptor 2 (HER2)) remain a major cause of breast cancer mortality because of their invasiveness and metastatic potential, and the lack of suitable molecular targets for treatment [8] , [9] . These tumours also show increased resistance to conventional chemotherapeutic agents. Hence, there is an urgent need to develop new therapeutic drugs that are effective against TNBCs and metastatic breast cancers (MBCs), especially those that can offer higher survival rates, fewer side effects and a better quality of life for patients than the currently available therapies. Oncogene addiction, a phenomenon that the survival of cancer cells depends on an activated oncogene, has been suggested as one of the major mechanisms underlying cancer progression and metastasis; targeting oncogenes has great potential for cancer treatment and prevention. Recent advances in breast cancer biology have demonstrated that the loss of tumour suppressors, such as p53 (ref. 10 ), and overexpression of oncogenes, including Mouse Double Minute 2 (MDM2; ref. 11 ), contribute to the poor response to treatment and poor prognosis in breast cancer patients, especially in TNBC, providing novel molecular targets for developing breast cancer therapies, especially for advanced disease. The MDM2 oncogene is amplified and overexpressed in a number of human malignancies, including breast cancer [12] , [13] , [14] , [15] . High levels of the MDM2 protein often correlate with decreased survival in patients [13] , [15] . The MDM2 oncogene is a negative regulator of the tumour suppressor p53, which regulates the cell cycle, maintains the genomic integrity of cells and controls the cellular response to DNA damage [16] , [17] . It also directly binds to p53 and represses the transcriptional activity of p53 (refs 16 , 17 ) and promotes p53 degradation [18] , [19] . The MDM2 oncoprotein also has p53-independent activities [15] , [20] . In addition to inhibiting apoptosis by affecting both pro-apoptotic and anti-apoptotic proteins [21] , [22] , MDM2 also alters cell cycle regulation, DNA replication and DNA repair [23] , [24] . Both animal studies with transgenic mice and clinical observations have established that MDM2 is involved in cancer development and the response to treatment, both dependent and independent of p53 (refs 25 , 26 ). We and others have suggested that MDM2 could be used as a target for cancer therapy and prevention and have provided evidence supporting this notion [27] , [28] , [29] , [30] . Thus far, most MDM2 inhibitors have been designed to block the MDM2–p53 binding, such as nutlin-3 (ref. 31 ), RITA [32] and MI219 (ref. 33 ). Such inhibition requires wild-type p53 expression in cancer cells [34] , [35] . Considering that the majority (50–75%) of breast cancers harbour mutant p53 and have high levels of MDM2, these MDM2 inhibitors are expected to have low or no efficacy against these types of breast cancer [36] . Therefore, it is highly desirable to design novel MDM2 inhibitors that have direct effects on MDM2 and exert their anticancer activity independent of the p53 status. In our continued efforts to develop novel MDM2 inhibitors, we show here that using a high-throughput virtual screening and structure-based drug design, we identified a series of pyrido[b]indole derivatives as highly selective MDM2 inhibitors. Among more than 200 MDM2-interative compounds synthesized, we selected and synthesized the 45 top candidates with excellent binding capacity to MDM2, followed by a sensitive, specific, cell-based screening for their in vitro anticancer activity. Among these compounds, one small molecule, named SP-141 (6-methoxy-1-(naphthalen-1-yl)-9 H-pyrido[3,4- b ]indole; Fig. 1a ) shows strong binding to the MDM2 protein and potent in vitro activity against several human breast cancer cell lines, regardless of p53 status. It inhibits MDM2 expression and promotes MDM2 autoubiquitination and proteasomal degradation. Furthermore, SP-141 decreases the tumour growth and inhibits metastasis in vivo . We believe that the present results provide a basis for the development of SP-141 as a novel therapeutic agent for breast cancer. 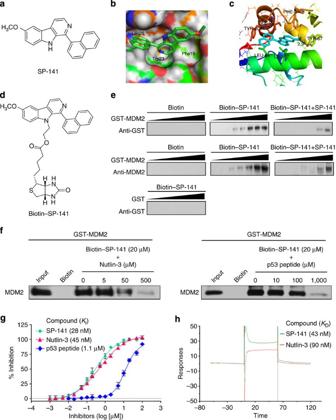Figure 1: SP-141 directly binds to the MDM2 protein. (a) The chemical structure of SP-141. (b) The binding site and orientation of SP-141 in the hydrophobic groove of MDM2. The protein is rendered as surface; SP-141 is rendered in green. (c) A model of the interaction of SP-141 with MDM2. MDM2 is rendered in cartoon form, while the residues in contact with SP-141 are rendered as sticks. The compound is coloured light blue. (d) The chemical structure of biotinylated SP-141. (e) Purified GST-MDM2 was incubated at various concentrations with biotinylated SP-141, which was then incubated with avidin beads in the presence or absence of 20 μM of non-biotinylated SP-141. Purified GST was used as a negative control. The bound protein was detected using anti-MDM2 and anti-GST antibodies. (f) Purified GST-MDM2 was incubated with biotinylated SP-141 (20 μM) that was incubated with avidin beads in the presence or the absence of Nutlin-3 (0, 5, 50 and 500 μM) and a natural p53 peptide (residues 16–27; 0, 10, 100 and 1,000 μM). The bound protein was detected using anti-MDM2 antibody. (g) Competitive binding to recombinant human MDM2 proteins using FP-based binding assay. Nutlin-3 and the natural p53 peptide were used as positive controls (mean±s.e.m.;n=9 for each data point). (h) CompetitiveKDvalues of SP-141 to MDM2 as determined using the Biacore assay. MDM2 protein was immobilized on a CM5 sensor chip. Nutlin-3 was used as a positive control. All assays were performed in triplicate, and all the experiments were repeated at least three times. Figure 1: SP-141 directly binds to the MDM2 protein. ( a ) The chemical structure of SP-141. ( b ) The binding site and orientation of SP-141 in the hydrophobic groove of MDM2. The protein is rendered as surface; SP-141 is rendered in green. ( c ) A model of the interaction of SP-141 with MDM2. MDM2 is rendered in cartoon form, while the residues in contact with SP-141 are rendered as sticks. The compound is coloured light blue. ( d ) The chemical structure of biotinylated SP-141. ( e ) Purified GST-MDM2 was incubated at various concentrations with biotinylated SP-141, which was then incubated with avidin beads in the presence or absence of 20 μM of non-biotinylated SP-141. Purified GST was used as a negative control. The bound protein was detected using anti-MDM2 and anti-GST antibodies. ( f ) Purified GST-MDM2 was incubated with biotinylated SP-141 (20 μM) that was incubated with avidin beads in the presence or the absence of Nutlin-3 (0, 5, 50 and 500 μM) and a natural p53 peptide (residues 16–27; 0, 10, 100 and 1,000 μM). The bound protein was detected using anti-MDM2 antibody. ( g ) Competitive binding to recombinant human MDM2 proteins using FP-based binding assay. Nutlin-3 and the natural p53 peptide were used as positive controls (mean±s.e.m. ; n =9 for each data point). ( h ) Competitive K D values of SP-141 to MDM2 as determined using the Biacore assay. MDM2 protein was immobilized on a CM5 sensor chip. Nutlin-3 was used as a positive control. All assays were performed in triplicate, and all the experiments were repeated at least three times. Full size image SP-141 is a specific MDM2 inhibitor By performing high-throughput virtual screening according to the published crystal structures of MDM2, a new class of pyrido[ b ]indole derivatives was discovered to have potent binding affinity for the MDM2 protein. On the basis of these core structures, we further designed a series of small molecule MDM2 inhibitors, and after initial cell-based screening, compound SP-141 was found to be the most active and was selected as a lead compound for further evaluation and development. A molecular modelling study of SP-141 and MDM2 was then carried out by using the docking software, Glide 2.5 (Schrodinger, New York, NY, USA). As shown in Fig. 1b,c , SP-141 occupied the Leu26 pocket and formed a hydrogen bond with Tyr-67. The naphthyl group of SP-141 could bind in the hydrophobic pocket occupied by Leu26 of p53, created by Leu54, Ile99, Tyr100 and Ile103 of MDM2. To obtain evidence supporting the specific binding of SP-141 to MDM2, we conjugated biotin to the 9-position nitrogen of SP-141 (see Supplementary Methods ). By performing a set of biotin-SP-141 pull-down assays using this newly synthesized biotin-SP-141 conjugate ( Fig. 1d ), we found that biotin-SP-141 specifically bound to MDM2, but not GST ( Fig. 1e ). Furthermore, this binding was significantly decreased, in a concentration-dependent manner, by the presence of unlabelled SP-141 ( Fig. 1e ), further confirming the specificity of the interaction between SP-141 and MDM2. We also determined whether Nutlin-3 and p53 peptides could block the binding of GST-MDM2 to Biotin-SP-141 in vitro . Our results showed that biotin-SP-141-MDM2 binding was markedly reduced by Nutlin-3 and a nature p53 peptide in a dose-dependent manner, indicating that SP-141 may occupy the p53-binding site on MDM2 ( Fig. 1f ). We further investigated the binding affinity of SP-141 to the MDM2 protein using a fluorescence polarization-based (FP-based) binding assay ( Fig. 1g ) and Biacore assay ( Fig. 1h ). The results from the FP-based assay demonstrated that SP-141 bound to MDM2 with a K i value of 28±6 nM, showing a significantly higher affinity than a nature p53 peptide (residues 16–27, K i =1.11±0.19 μM) and nutlin-3 ( K i =45±4 nM). In the Biacore assay, SP-141 also showed a better binding affinity to the MDM2 protein ( K D =43 nM) than the positive control, nutlin-3 ( K D =90 nM). Taken together, all these findings demonstrated that SP-141 was a specific MDM2 inhibitor with a high binding capacity for the MDM2 protein. SP-141 exerts cytotoxic effects on breast cancer cells SP-141 was evaluated for its effects on breast cancer cell viability in vitro using the 3-(4,5-dimethylthiazol-2-yl)-2,5-diphenyl tetrazolium bromide (MTT) assay. Five human breast cancer cell lines representing three different genetic backgrounds (MCF-7/p53 wild type (wt); MCF-7/p53 knockdown (KD), MDA-MB-468/p53 mutant (mt), MDA-MB-231/p53 mt and MDA-MB-435/p53 mt) and one ‘normal’ (immortalized but non-malignant) breast epithelial cell line (MCF-10A) were cultured with the compound at concentrations ranging from 0 to 25 μM for 72 h, and the cell viability was determined. The IC 50 (the concentration that inhibits the survival of cells by 50%) values were calculated following incubation with various concentrations of the compound ( Fig. 2a ). The compound had IC 50 values of less than 1 μM (0.39–0.91 μM) in human breast cancer cells. The MCF-10A cells were less sensitive (IC 50 : 11.74 μM) to the inhibitory effects of SP-141 than the breast cancer cells. SP-141 also inhibited cancer cell colony formation in a concentration-dependent manner ( Fig. 2b ). 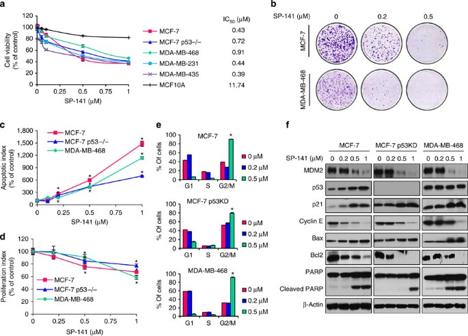Figure 2: SP-141 induces breast cancer cell death. Cells were exposed to various concentrations of SP-141 for (a) 72 h for the MTT assay to evaluate the cell viability and IC50value; (b) 24 h for the colony formation assay; (c) 48 h for the apoptosis assay; (d) 24 h for the proliferation assay; (e) 24 h for the cell cycle distribution assay or (f) 24 h before a western blot analysis of the expression of MDM2 and proteins related to apoptosis and cell cycle arrest in human breast cancer cells. All assays were performed in triplicate, and all the experiments were repeated at least three times (mean±s.e.m.,n=9 for each data point, two-sided Student’st-test, *P<0.01). Figure 2: SP-141 induces breast cancer cell death. Cells were exposed to various concentrations of SP-141 for ( a ) 72 h for the MTT assay to evaluate the cell viability and IC 50 value; ( b ) 24 h for the colony formation assay; ( c ) 48 h for the apoptosis assay; ( d ) 24 h for the proliferation assay; ( e ) 24 h for the cell cycle distribution assay or ( f ) 24 h before a western blot analysis of the expression of MDM2 and proteins related to apoptosis and cell cycle arrest in human breast cancer cells. All assays were performed in triplicate, and all the experiments were repeated at least three times (mean±s.e.m., n =9 for each data point, two-sided Student’s t- test, * P <0.01). Full size image To begin assessing the mechanism(s) by which the compound exerts its effects against breast cancer cells, we first examined its effects on cell apoptosis. As illustrated in Fig. 2c , all three of the examined breast cancer cell lines exhibited a significant concentration-dependent increase ( P <0.01) in apoptosis. In the p53 wt MCF-7, p53 KD MCF-7 and p53 mt MDA-MB-468 cells, a 1-μM concentration of SP-141 increased the apoptotic index 14-fold ( P <0.01), 7-fold ( P <0.01) and 11-fold ( P <0.01) higher than that seen in control cells, respectively. Similar to the effects on cell survival, SP-141 concentration-dependently inhibited cell proliferation ( Fig. 2d ) in all three human breast cancer cell lines. The MDA-MB-468 cells were more sensitive to SP-141 treatment at the highest concentration (1 μM) than were the MCF-7 and MCF-7 p53 KD cells. However, the MCF-7 cells (both p53 wt and p53 KD) were more sensitive to the lower concentrations of SP-141, with a 0.5-μM concentration leading to a significant decrease in proliferation ( P <0.01). SP-141 was also examined for effects on cell cycle progression ( Fig. 2e ). In all three cell lines, SP-141 significantly induced cell cycle arrest in the G2 phase at the 0.5 μM concentration ( P <0.01). The effects of SP-141 on MDM2 expression were analysed in all three breast cancer cell lines. As shown in Fig. 2f , the MDM2 protein levels were decreased in a concentration-dependent manner in all three cell lines. In the MCF-7 (p53 wt) cells, the wild-type p53 protein level was increased, most likely as a result of the inhibition of MDM2. In addition, the expression level of p21 Waf1/CIP1 , a MDM2 target gene, was also elevated in all three cell lines, likely as a result of MDM2 inhibition. We also assessed the expression of several apoptosis- and cell cycle-related proteins. Consistent with its effects on apoptosis and the cell cycle, SP-141 increased the expression of cleaved PARP and Bax and decreased the expression of Bcl-2 and Cyclin E in a p53-independent manner. SP-141 inhibits xenograft tumour growth in vivo To determine whether the compound was effective against tumours growing in vivo , SP-141 was administered to nude mice bearing MCF-7 and MDA-MB-468 xenograft tumours. SP-141 was administered by intraperitoneal (i.p.) injection at doses of 40 mg kg −1 per day for 42 and 30 days, respectively. As shown in Fig. 3a–d , SP-141 inhibited the MCF-7 and MDA-MB-468 xenograft tumour growth by ~82% ( P <0.01) on day 42 ( Fig. 3a,c ), and ~80% ( P <0.01) on day 30 ( Fig. 3b,d ), respectively. In addition, no significant host toxicity was observed at this dose in either model, as monitored by changes in body weight ( Fig. 3e,f ). There were also no gross organ (liver, lung, kidney, spleen, heart or brain) abnormalities at necropsy in the treatment group noted during histological examinations in the mice bearing MCF-7 xenograft tumours ( Fig. 3g ). 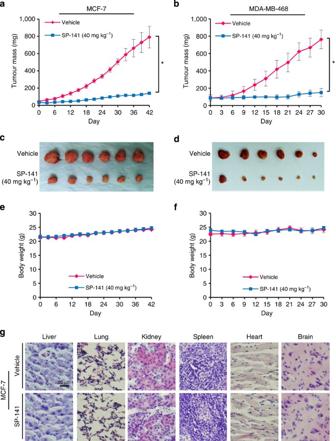Figure 3: SP-141 suppresses breast xenograft tumour growthin vivo. Nude mice bearing MCF-7 (a) and MDA-MB-468 (b) xenograft tumours were treated with SP-141, which was administered by i.p. injection at 40 mg kg−1per day, 5 d per week for 42 and 30 days, respectively. (c,d) At the end of the experiments, representative tumours were removed and photographed. Animals were also monitored for changes in body weight as a surrogate marker for toxicity in both the MCF-7 (e) and MDA-MB-468 (f) xenograft models. (g) At the termination of the experiments, H&E staining of the paraffin sections of some organs from mice bearing MCF-7 xenograft tumours was performed (scale bar, 20 μm). (Mean±s.e.m.,n>10 for each data point, two-sided Student’st-test, *P<0.01). Figure 3: SP-141 suppresses breast xenograft tumour growth in vivo . Nude mice bearing MCF-7 ( a ) and MDA-MB-468 ( b ) xenograft tumours were treated with SP-141, which was administered by i.p. injection at 40 mg kg −1 per day, 5 d per week for 42 and 30 days, respectively. ( c , d ) At the end of the experiments, representative tumours were removed and photographed. Animals were also monitored for changes in body weight as a surrogate marker for toxicity in both the MCF-7 ( e ) and MDA-MB-468 ( f ) xenograft models. ( g ) At the termination of the experiments, H&E staining of the paraffin sections of some organs from mice bearing MCF-7 xenograft tumours was performed (scale bar, 20 μm). (Mean±s.e.m., n >10 for each data point, two-sided Student’s t- test, * P <0.01). Full size image To further validate the molecular mechanism(s) underlying the effects of SP-141, we further evaluated the expression levels of the various apoptosis- and cell cycle-related proteins in vivo ( Fig. 4 ). As shown in Fig. 4a , the protein levels of MDM2 were reduced and those of p53 were increased in the MCF-7 xenograft tumours, as determined with immunohistochemical staining. To confirm these observations, western blot analyses were performed, and consistent with the in vitro data, the protein levels of MDM2 were decreased by SP-141, resulting in elevated expression of p53, p21, Bax and cleaved PARP and decreased expression of Cyclin E and Bcl-2 ( Fig. 4b ). Similar results were seen in the MDA-MB-468 xenograft model ( Fig. 4c ). 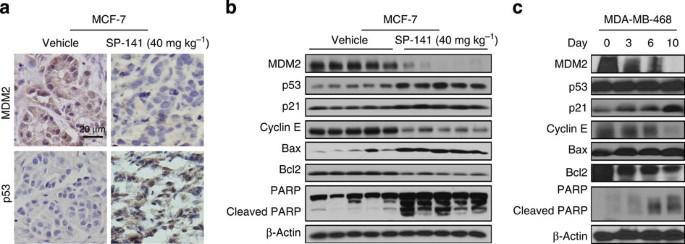Figure 4: SP-141 decreases the MDM2 expressionin vivo. Nude mice bearing MCF-7 and MDA-MB-468 xenograft tumours were treated with SP-141, which was administered by i.p. injection at 40 mg kg−1per day, 5 day per week for 42 and 30 days, respectively. At the end of the experiment, MCF-7 xenograft tumours were removed and further analysed for their protein expression with immunohistochemistry (scale bar, 20 μm;a) and western blotting (each lane represents a different tumour sample;b). (c) On different days (0, 3, 6 and 10), MDA-MB-468 xenograft tumours were homogenized and analysed with western blot analysis. All the experiments were repeated at least three times. Figure 4: SP-141 decreases the MDM2 expression in vivo. Nude mice bearing MCF-7 and MDA-MB-468 xenograft tumours were treated with SP-141, which was administered by i.p. injection at 40 mg kg −1 per day, 5 day per week for 42 and 30 days, respectively. At the end of the experiment, MCF-7 xenograft tumours were removed and further analysed for their protein expression with immunohistochemistry (scale bar, 20 μm; a ) and western blotting (each lane represents a different tumour sample; b ). ( c ) On different days (0, 3, 6 and 10), MDA-MB-468 xenograft tumours were homogenized and analysed with western blot analysis. All the experiments were repeated at least three times. Full size image Taken together, these data suggest that SP-141 effectively suppresses the growth of breast cancer xenograft tumours. SP-141 induces MDM2 protein degradation To elucidate the possible mechanism(s) responsible for the SP-141-induced MDM2 inhibition in vitro and in vivo , we treated breast cancer cells with 0.5 μM of SP-141 or vehicle control for 24 h, followed by exposure to the protein synthesis inhibitor, cycloheximide (15 μg ml −1 ) for various times. As shown in Fig. 5a , SP-141 increased the degradation rate of the MDM2 protein in both MCF-7 and MDA-MB-468 cells. The p53 protein was stabilized in MCF-7 cells, but not in the p53 mt MDA-MB-468 cells. 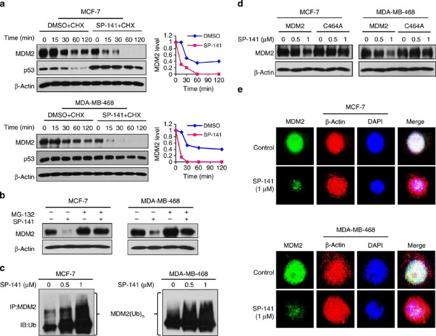Figure 5: SP-141 destabilizes the MDM2 protein. (a) MCF-7 and MDA-MB-468 cells were treated with SP-141 (0.5 μM), and then exposed to cycloheximide (CHX, 15 μg ml−1), an inhibitor of protein synthesis. The MDM2 protein levels were detected with western blot analysis. The graphs on the right show the quantification of the western blot data. (b) Cells were treated with SP-141 (0.5 μM) for 24 h, and then were exposed to a proteasome inhibitor, MG 132 (25 μM), for an additional 6 h. The protein levels of MDM2 were detected with western blot analysis. (c) Cells were transfected with MDM2 and ubiquitin plasmids, followed by treatment with SP-141 for 24 h. The cells were then exposed to MG132 (25 μM) for an additional 6 h, and the lysates were subjected to immunoprecipitation with an MDM2 antibody. The ubiquitinated MDM2 was detected using an antiubiquitin antibody. (d) Cells were transfected with a wild-type MDM2 plasmid or mutant MDM2 plasmid without E3 ligase activity (C464A). After treatment with SP-141 for 24 h, and MDM2 levels were detected with western blot analysis. (e) Representative images of MDM2 immunofluorescence in control and SP-141 (1 μM)-treated cells. β-actin and DAPI were used as internal references. All the experiments were repeated three times. Figure 5: SP-141 destabilizes the MDM2 protein. ( a ) MCF-7 and MDA-MB-468 cells were treated with SP-141 (0.5 μM), and then exposed to cycloheximide (CHX, 15 μg ml −1 ), an inhibitor of protein synthesis. The MDM2 protein levels were detected with western blot analysis. The graphs on the right show the quantification of the western blot data. ( b ) Cells were treated with SP-141 (0.5 μM) for 24 h, and then were exposed to a proteasome inhibitor, MG 132 (25 μM), for an additional 6 h. The protein levels of MDM2 were detected with western blot analysis. ( c ) Cells were transfected with MDM2 and ubiquitin plasmids, followed by treatment with SP-141 for 24 h. The cells were then exposed to MG132 (25 μM) for an additional 6 h, and the lysates were subjected to immunoprecipitation with an MDM2 antibody. The ubiquitinated MDM2 was detected using an antiubiquitin antibody. ( d ) Cells were transfected with a wild-type MDM2 plasmid or mutant MDM2 plasmid without E3 ligase activity (C464A). After treatment with SP-141 for 24 h, and MDM2 levels were detected with western blot analysis. ( e ) Representative images of MDM2 immunofluorescence in control and SP-141 (1 μM)-treated cells. β-actin and DAPI were used as internal references. All the experiments were repeated three times. Full size image To elucidate the underlying mechanisms, the breast cancer cells were treated with MG132 (25 μM), a proteasome inhibitor. This treatment reduced the effects of SP-141 on MDM2 ( Fig. 5b ), suggesting that the SP-141-induced MDM2 degradation is proteasome-dependent. Co-treatment with MG132 also showed that SP-141 increased MDM2 ubiquitination with immunoprecipitation assay ( Fig. 5c ). MDM2 harbours a self-targeting E3 ubiquitin ligase, and its protein degradation is regulated by its autoubiquitination activity [37] . We therefore next elucidated whether SP-141 induces MDM2 autoubiquitination. To accomplish this, cells were transfected with MDM2 or an MDM2 mutant (C464A) without E3 ubiquitin ligase activity. As shown in Fig. 5d , the amount of wild-type MDM2 was decreased by SP-141, while the mutant MDM2 was resistant to the degradation induced by SP-141. The downregulation of MDM2 by SP-141 was further confirmed by an immunofluorescence study. Compared with the control cells, the MDM2 staining was markedly decreased in SP-141-treated cells in both cell lines ( Fig. 5e ). MDM2 KD blocks the inhibitory effects of SP-141 To confirm that the antibreast cancer activity of SP-141 is dependent on its effects on MDM2, we compared the effects of SP-141 on parent and inducible MDM2 KD MCF-7 cells. As shown in Fig. 6 , Tet treatment resulted in ~79% KD of MDM2 protein expression ( Fig. 6a ). MDM2 KD itself inhibited colony formation ( Fig. 6b ) and increased apoptosis ( Fig. 6c ). After SP-141 treatment, compared with the parent cells, MDM2 KD reduced the effects of SP-141 on the MDM2 protein degradation ( Fig. 6a ) and reversed the cellular responses to SP-141, including the decrease in colony formation ( Fig. 6b ) and increase in apoptosis ( Fig. 6c ), indicating a critical role for MDM2 in the SP-141-induced growth inhibition of breast cancer cells. 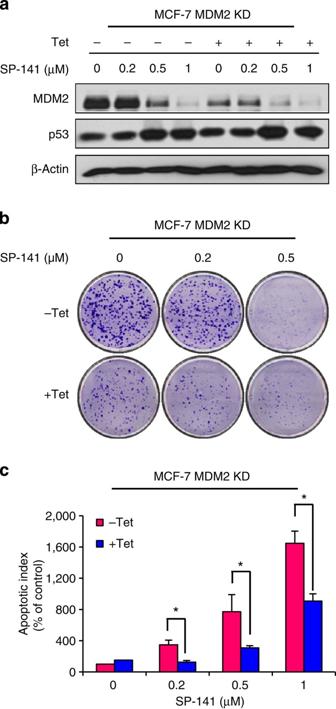Figure 6: MDM2 KD reduces the inhibitory effects of SP-141. Inducible MDM2 KD MCF-7 cells were incubated with (+Tet; 1 μg ml−1) or without (−Tet) tetracycline for 24 h, followed by exposure to various concentrations of SP-141 (0–1 μM) for various times: (a) 24 h for the expression of proteins; (b) 24 h for the colony formation assay; and (c) 48 h for the apoptosis assay. All assays were performed in triplicate, and all the experiments were repeated at least three times. (Mean±s.e.m.,n=9 for each data point, two-sided Student’st-test, *P<0.01). Figure 6: MDM2 KD reduces the inhibitory effects of SP-141. Inducible MDM2 KD MCF-7 cells were incubated with (+Tet; 1 μg ml −1 ) or without (−Tet) tetracycline for 24 h, followed by exposure to various concentrations of SP-141 (0–1 μM) for various times: ( a ) 24 h for the expression of proteins; ( b ) 24 h for the colony formation assay; and ( c ) 48 h for the apoptosis assay. All assays were performed in triplicate, and all the experiments were repeated at least three times. (Mean±s.e.m., n =9 for each data point, two-sided Student’s t- test, * P <0.01). Full size image SP-141 inhibits cell migration in vitro and in vivo MBC is responsible for the majority of breast cancer deaths. Currently, the 5-year overall survival rate for MBC is less than 25% (ref. 38 ). A crucial component of tumour cell invasion is cell migration. To investigate the effects of SP-141 on cancer cell motility, the wound-healing assay was performed using MDA-MB-231 human breast cancer cells. The cells were treated with the vehicle, or with 0.1 or 0.2 μM of SP-141, and the cell migration into the wound made in the cell monolayer was evaluated. As shown in Fig. 7a , the control cells readily closed the wound over a period of 20 h. The SP-141 treatment significantly decreased the cell migration in a concentration-dependent manner from 4 to 20 h in various breast cancer cell lines. 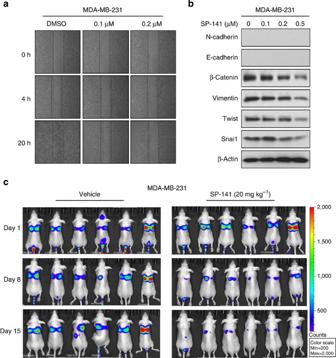Figure 7: SP-141 inhibits cell metastasisin vitroandin vivo. (a) MDA-MB-231 cells were grown to confluence in a six-well plate and a scratch was made at experimental time zero, and then the cells were exposed to various concentrations of SP-141. The wells were imaged at different time points. All the experiments were repeated at least three times. (b) The effects of SP-141 on the expression of EMT-related proteins in MDA-MB-231 cells. All the experiments were repeated at least three times. (c) About 1 × 106MDA-MB-231-Luc cells were intravenously injected into a tail vein of nude mice. SP-141 was administered by i.p. injection at doses of 20 mg kg−1per day, 5 days per week for 2 weeks. The luciferase signals in the mice were detected and photographed using an IVISin vivoimage system on days 1, 8 and 15. Figure 7: SP-141 inhibits cell metastasis in vitro and in vivo . ( a ) MDA-MB-231 cells were grown to confluence in a six-well plate and a scratch was made at experimental time zero, and then the cells were exposed to various concentrations of SP-141. The wells were imaged at different time points. All the experiments were repeated at least three times. ( b ) The effects of SP-141 on the expression of EMT-related proteins in MDA-MB-231 cells. All the experiments were repeated at least three times. ( c ) About 1 × 10 6 MDA-MB-231-Luc cells were intravenously injected into a tail vein of nude mice. SP-141 was administered by i.p. injection at doses of 20 mg kg −1 per day, 5 days per week for 2 weeks. The luciferase signals in the mice were detected and photographed using an IVIS in vivo image system on days 1, 8 and 15. Full size image The epithelial–mesenchymal transition (EMT) is defined by the loss of epithelial characteristics and the acquisition of a mesenchymal phenotype. The EMT produces cancer cells that are invasive, migratory and exhibit stem cell characteristics, hallmarks of cells that have metastatic potential [39] , [40] . To gain insight into the role of SP-141 in cell migration, we investigated whether the decreased migration of cells treated with SP-141 resulted in the inhibition of EMT-related molecular markers. The results demonstrated that treatment of the cells with SP-141 for 24 h led to concentration-dependent decreases in the expression of β-catenin, vimentin, Twist and Snai1 ( Fig. 7b ). To validate the antimetastatic effects of SP-141 in vivo , we performed experimental metastasis assays. MDA-MB-231-Luc breast cancer cells were intravenously injected into a tail vein of nu/nu mice. The animals were randomly divided into a treatment group and a control group after cell injection. SP-141 was administered by i.p injection at doses of 20 mg kg −1 per day for 2 weeks. As determined using the IVIS in vivo imaging system, the MDA-MB-231-Luc illumination signals in the lung tissues of control mice were significantly stronger than those in the SP-141-treated mice on Days 8 and 15 ( Fig. 7c ), indicating that the SP-141 treatment decreased the metastasis of breast cancer cells. There is an increasing interest in developing MDM2 inhibitors as novel anticancer agents. In our pursuit of small molecule MDM2 inhibitors, we discovered a series of pyrido[ b ]indole derivatives with strong binding affinity for the MDM2 protein and the ability to influence the MDM2 levels, regardless of the p53 status. On the basis of initial screening studies, SP-141 was chosen as a lead compound because of its excellent in vitro activity against breast cancer. The present study was the first to investigate both the in vitro and in vivo antitumour effects of the novel pyrido[ b ]indole compound in human breast cancer cell lines. We have demonstrated several important points. First, SP-141 is a novel computer-designed MDM2 inhibitor that directly targets the MDM2 protein. Second, SP-141 significantly inhibits breast cancer cell growth, but with much lower activity in normal cells, indicating its specificity for cancer cells. SP-141 also reduces the breast cancer cell colony formation, inhibits cell proliferation, induces apoptosis and arrests cells in the G2/M phase, regardless of their p53 status. Third, SP-141 downregulates MDM2 expression and destabilizes the MDM2 protein by promoting its ubiquitination in vitro , regardless of the p53 status of the cells. Fourth, SP-141 decreases the growth of tumours in two different breast cancer xenograft models and inhibits the MDM2 expression and modulates the protein levels of various other proteins, with changes similar to those observed in vitro , independent of the p53 status. Fifth, the inhibition of MDM2 by SP-141 is essential for its antitumour activities. Finally, SP-141 inhibits breast cancer cell migration in vitro and metastasis in vivo . These results demonstrated that SP-141 is an effective therapeutic agent that may have potential for the treatment of human breast cancer. The present findings clearly indicated that SP-141 exerts its antibreast cancer activity by directly targeting MDM2, inducing MDM2 degradation, regardless of the p53 status of the cells. Also of note, we did not observe any significant toxicity (as indicated by the histological examination of various tissues and by the body weight changes) in the mice. This is remarkable because these studies were performed after 6 weeks of treatment at a relatively high dose of 40 mg kg −1 per day. It is possible that by further optimizing the dosing frequency or formulation, might be possible to achieve significant anticancer activity at lower doses. In the present study, we showed that SP-141 specifically bound to the MDM2 protein, based on the results from several assays, including the initial molecular docking, biotin–avidin pull-down assays, FP-based binding assay and Biacore assay. We demonstrated that SP-141 significantly decreased the growth of cancer cells with both wild-type (MCF-7) and non-functional (MCF-7 p53 KD, MDA-MB-468) p53, as well as oestrogen receptor-dependent (MCF-7) and -independent (MDA-MB-468) cancer cells. To confirm the activity of the compound, we also investigated its in vivo effects. SP-141 decreased the growth of both MCF-7 and MDA-MB-468 xenograft tumours. Most important, we demonstrated that the downregulation of the MDM2 oncoprotein is responsible for the observed cytotoxic effects of SP-141. It is known that MDM2 possesses E3 ubiquitin ligase activity, and that its degradation largely depends on autoubiquitination [37] . Our results indicated that SP-141 destabilized the MDM2 protein by promoting its autoubiquitination and proteasomal degradation, a unique molecular mechanism of action different from all of the existing MDM2 inhibitors; however, it remains largely unknown how SP-141 causes MDM2 rapid autoubiquitination and degradation. Today, it is known that E3 ubiquitin ligases play key roles in cellular processes and functions, and dimerization is required for some E3s activity [41] . For instance, smac mimetic compounds, a novel class of small molecule antagonists, sensitize cells to apoptosis by targeting the inhibitor of apoptosis (IAP) proteins. The binding of smac mimetic compounds to cIAPs results in conformational rearrangements of cIAPs, promoting its RING domain dimerization, leading to the autoubiquitination and proteasomal degradation of cIAPs [42] , [43] . We also have determined whether SP-141can cause any aggregation (for example, dimerization) of MDM2 using gluteraldehyde crosslink assay. MDM2 formed oligomers in both MCF-7 and MDA-MB-468 cells, and MDM2 oligomer formation was not changed at any concentrations of SP-141, suggesting that aggregation may not be the reason for SP-141 to cause rapid autoubiquitination and degradation of MDM2. Further detailed analysis and investigations are required to identify the mechanisms. In target validation, a withdrawal of the interested target (using short interfering RNA or short hairpin RNA or DNA deletion of the target gene to remove the drug target) is the commonly used technique. In most cases, loss of the target results in less sensitivity to the drug or even resistance to the drug. Knockdown of MDM2 has been used to demonstrate the specificity of the test drugs [44] , [45] . In the present study, in order to validate that MDM2 is the major target of SP-141, we used Tet-On tetracycline-inducible expression systems and confirmed that KD of MDM2 resulted in the inhibition of cell growth and induction of apoptosis and that the MDM2 KD cells were resistant to the compound, showing less sensitivity in terms of the cell colony formation and apoptosis. The loss of sensitivity is most likely due to the loss of molecular target (MDM2). These results indicated the importance of MDM2 inhibition in the SP-141-induced antibreast cancer activities. These results also indicated that the SP-141-MDM2 complex was needed for its cytotoxicity against cancer cells. However, in the present study, there was still no sufficient evidence supporting a direct link between binding of SP-141 and its ability to induce MDM2 degradation. In future studies, additional techniques such as protein mutation, gene knockout, pharmacological inhibitors and transgenic mouse models should be employed to generate more direct evidence for establishing the direct link between SP-141–MDM2 binding, MDM2 degradation and anticancer activity. MDM2 overexpression may be responsible for the drug resistance and radio resistance of human cancer cells, and may be associated with tumour invasion, high-grade/late-stage tumours, tumour recurrence and metastasis, and is a negative prognostic factor for cancer patients [36] , [46] , [47] . In this study, we provide compelling evidence from cell and animal studies that, in addition to its effects on the primary tumour, SP-141 also has antimetastatic effects. We demonstrated that SP-141 repressed the migration of MDA-MB-231 cells. In addition, SP-141 treatment altered the expression levels of EMT-related proteins that are involved in crucial metastasis pathways, such as β-catenin, vimentin, Twist and Snai1. The results of our in vivo experimental metastasis assays confirmed that SP-141 suppressed tumour metastasis, likely through the inhibition of cell migration. We propose that SP-141 can inhibit tumour cell metastasis at least partly through its inhibition of MDM2 activity. Taken together, these results indicate that SP-141 exerted its effects primarily by inhibiting cancer cell growth, colony formation, proliferation, cell cycle progression and migration. SP-141 exerts these effects and also induces apoptosis by targeting MDM2, making use of both p53-dependent and -independent, as well as ER-dependent and -independent pathways. In summary, considering the important role of MDM2 in cancer growth and progression, we speculate that SP-141 can be developed as a novel small molecule that can serve as a molecular-targeted chemotherapeutic agent. The results of the present study provide initial critical information regarding the efficacy and safety of the compound, and on the value of directly targeting MDM2 for breast cancer therapy. Molecular modelling The initial virtual screening was carried out using the first reported MDM2-p53 complex crystal structure (PDB ID 1YCR) [48] , which led to the identification of the pyrido[ b ]indole scaffold, on which further structures were designed and synthesized. A more recent docking study was undertaken with a refined structure of MDM2 (PDB: 4ERE) using the Maestro 9.0 software programme (Schrodinger). All water molecules were removed from the complex structure, and the hydrogen atoms and charges were added during a brief relaxation performed using the ‘Protein Preparation Wizard’ workflow in the Maestro 9.0 programme. After optimizing the hydrogen bond network, the crystal structure was minimized using the OPLS 2005 force field, with the maximum RMSD value set at 0.3 Å. The grid box was centred on the ligand AM-8553 in the crystal structure, as described above, and was defined so as to enclose residues located within 14 Å from the ligand. A scaling factor of 1.0 was set to van der Waals radii, with the partial atomic charges scaled by 0.25 to soften the nonpolar parts of the receptor. The three-dimensional structures of the compound were generated using the Ligprep module. Extra precision docking approaches were adopted successively. Synthesis and purification of the test compound The 5-methoxy tryptamine (0.524 mM) and 1-naphthaldehyde (0.63 mM) were dissolved in anhydrous tetrahydrofuran (20 ml). The reaction mixture was cooled to 0 ° C, and trifluoroacetic acid (CF 3 COOH, 0.2 ml) was then added dropwise at 0 °C. The reaction mixture was allowed to stir at 0 °C for 1 h, and the ice bath was then removed and the reaction mixture was stirred for another hour. The mixture was quenched with an aqueous saturated solution of sodium bicarbonate (NaHCO 3 , 5 ml) and the organic phase was separated. The mixture was extracted with ethyl acetate (2 × 10 ml). The combined organic phase was dried over anhydrous sodium sulfate (Na 2 SO 4 ), filtered and evaporated under reduced pressure to give the crude tetrahydro-β-carboline intermediate product. The tetrahydro-β-carboline intermediate was used for the second step to oxidize it to the full β-carboline target product as follows: To a solution of the tetrahydro-β-carboline product in anhydrous xylene (10 ml) 10% Pd/C (50–100 mg) was added, and the mixture was refluxed for 10 h. The reaction mixture was then cooled and filtered through celite and washed with methanol (5–10 ml). Evaporation of the xylene/MeOH filtrate under reduced pressure yielded a crude product. The crude product was subjected to flash silica gel chromatography eluting with a 5% methanol–dichloromethane mixture to obtain the pure β-carboline target product, SP-141, which was characterized by its melting point, infrared spectroscopy, mass spectrometry, high-resolution nuclear magnetic resonance and an elemental analysis. Binding of biotinylated SP-141 to the MDM2 protein in vitro The preparation and purification of the recombinant GST and GST-MDM2 proteins were described previously [49] . Biotin- or biotin-SP-141-conjugated agarose beads were prepared as reported previously [50] . Briefly, recombinant GST or GST-MDM2 proteins were incubated with biotin or biotin-SP-141 beads in the absence or presence of unlabelled SP-141 (20 μM), or nutlin-3 (5, 50 and 500 μM), or a natural p53 peptide (residues 16–27, QETFSDLWKLLP-NH2; 10, 100 and 1,000 μM) overnight at 4 °C, and the bead-bound proteins were separated with SDS–PAGE and immunoblotted with anti-MDM2 and anti-GST antibodies. The details are provided in the Supplementary Methods . FP competitive binding assay Briefly, serial dilutions of the tested compound SP-141, nutlin-3, a natural p53 peptide (residues 16–27) with detergent (Tween 20, 0.005%, to reduce possible aggregation of hydrophobic inhibitors) and the assay buffer (100 mM potassium phosphate, pH 7.5; 100 μg ml −1 bovine gamma globulin; and 0.02% sodium azide) with pre-incubated MDM2 protein (10 nM, GST-MDM2) and PMDM6-F peptide (1 nM) were added in Dynex 96-well black, round-bottom plates, and the FP values were measured after a 3-h incubation. For each assay, the controls included the MDM2 protein and PMDM6-F (equivalent to 0% inhibition) and only PMDM6-F peptide (equivalent to 100% inhibition). The binding affinity constant ( K i ) of the test compound was calculated using a web-based computer programme ( http://sw16.im.med.umich.edu/software/calc_ki/ ) [51] , [52] . Biacore assay The Biacore assay was performed on a Biacore T-200 instrument at 25 °C using 10 mM HEPES buffer (pH 7.4), 150 mM NaCl, 3 mM EDTA, 0.005% P20 (polyoxyethylenesorbitan) and 5% dimethylsulphoxide (DMSO) as running buffer with a constant flow rate of 30 μl min −1 . His-MDM2 (1–118; Abcam Inc, USA) in 10 mM sodium acetate buffer (pH 4.5) was captured on flow cell 2, coated with anti-His antibody [31] . Gradient concentrations of SP-141 (0~10 μM) and nutlin-3 (0~10 μM) dissolved in the running buffer were streamed over the chip. Binding of analyst to the ligand was monitored in real time. The equilibrium constant ( K D ) was calculated using steady-state kinetics. Chemicals, plasmids and reagents All chemicals and solvents used were of the highest analytical grade available. Cell culture supplies and media, including PBS, sodium pyruvate, non-essential amino acids and penicillin–streptomycin, were obtained from Invitrogen (Carlsbad, CA, USA). Fetal bovine serum (FBS) was also obtained from Invitrogen. The anti-human Bax (N-20; 1:1,000), Bcl-2 (100; 1:1,000), MDM2 (SMP14; 1:500), PARP1 (H-250; 1:1,000), p21 (C19; 1:1,000), β-catenin (12F7; 1:2,000), Twist (Twist2C1a; 1:1,000) and Snai1 (G-7; 1:1,000) antibodies were from Santa Cruz Biotechnology Inc. (Santa Cruz, CA, USA). The anti-human p53 (Ab-6; 1:1,000) antibody was from EMD Chemicals Inc. (Gibbstown, NJ, USA). The anti-human N-cadherin (32/N-Cadherin; 1:1,000) and E-cadherin (36/E-Cadherin; 1:1,000) antibodies were from BD Biosciences (San Jose, CA, USA), and the anti-human vimentin (V9; 1:1,000) antibody was from Sigma-Aldrich Co. (St Louis, MO, USA). The anti-GST (GST01; 1:2,000) antibody was from ThermoFisher Scientific (Pittsburgh, PA, USA). Cell lines and culture Human breast cancer and non-malignant epithelial cells were obtained from the American Type Culture Collection (Rockville, MD, USA). MDA-MB-231 cells stably expressing luciferase (MDA-MB-231-Luc) were obtained from Caliper Lifesciences (Hopkinton, MA, USA). All cell culture media contained 10% FBS and 1% penicillin–streptomycin unless otherwise specified. Human MCF-7, MDA-MB-231 and MDA-MB-435 cells were grown in DMEM media. The MCF-7 p53 KD and MCF-7 MDM2 KD inducible cells were generated using the previously described method [53] , [54] and were grown in the same media as MCF-7 cells, but supplemented with 0.5 μg ml −1 puromycin or 10 μg ml −1 blasticidin and 0.5 μg ml −1 puromycin (Sigma-Aldrich Co.), respectively. MDA-MB-468 cells were grown in DMEM/F-12 Ham’s media (DMEM/F-12 1:1 mixture). The MCF-10A growth medium was composed of DMEM/F-12, supplemented with 5% donor horse serum, 20 ng ml −1 epidermal growth factor, 10 μg ml −1 insulin, 0.5 μg ml −1 hydrocortisone (Sigma-Aldrich Co.) and 100 ng ml −1 cholera toxin (Cambrex, Westborough, MA, USA). Human MDA-MB-231-Luc cells were grown in DMEM media containing 0.1 mM MEM non-essential amino acids and 2 mM L -glutamine. Analyses of cytotoxic effects The effects of the test compound on human breast cancer cell growth and viability, expressed as the percentage of cell survival, were determined using the MTT assay as described previously [54] , [55] , [56] . Cells were grown in 96-well plates at 3–4 × 10 3 cells per well, and were exposed to the test compound (0–25 μM) for 72 h. After incubation with the compound, 10 μl of the MTT solution (5 mg ml −1 ; Sigma-Aldrich Co.) were added to each well. The plates were incubated for 2–4 h at 37 °C. The supernatant was then removed, and the formazan crystals were dissolved in 100 μl of DMSO. The absorbance at 570 nm was recorded using a SYNERGY Mx microplate reader (BioTek, Winooski, VT, USA). The cell survival percentages were calculated by dividing the mean OD of compound-containing wells by that of DMSO-treated control wells. The effects of SP-141 on cell proliferation were determined using the BrdUrd incorporation assay (Oncogene, La Jolla, CA, USA) as reported previously [54] , [55] , [56] . In brief, cells were seeded in 96-well plates (3–5 × 10 3 cells per well) and incubated with various concentrations of SP-141 (0, 0.1, 0.2, 0.5 and 1 μM) for 24 h. BrdUrd was added to the medium 10 h before termination of the experiment. The BrdUrd incorporated into cells was determined using an anti-BrdUrd antibody, and the absorbance was measured at dual wavelengths of 450/540 nm using a SYNERGY Mx microplate reader (BioTek). Cells in early and late stages of apoptosis were detected using an Annexin V-FITC apoptosis detection kit from BioVision (Mountain View, CA, USA) according to the manufacturer’s protocol, as described previously [54] , [55] , [56] . In this procedure, 2–3 × 10 5 cells were exposed to the test compound (0, 0.2, 0.5 and 1 μM) and incubated for 48 h before the analysis. Cells were collected and washed with serum-free media, then resuspended in 500 μl of Annexin V binding buffer, followed by the addition of 5 μl of Annexin V-FITC and 5 μl of propidium iodide. The samples were incubated in the dark for 5 min at room temperature and were analysed with a FACSCaliber flow cytometer (BD Biosciences). To determine the effects of the compound on the cell cycle distribution using the method described previously [54] , [55] , [56] , cells (2–3 × 10 5 per well) were exposed to the test compound (0, 0.2 or 0.5 μM) and incubated for 24 h before the analysis. The cells were then trypsinized, washed with PBS and fixed in 1.5 ml of 95% ethanol at 4 °C overnight, followed by incubation with RNAse and staining with propidium iodide (Sigma-Aldrich Co.). The DNA content was determined using flow cytometry. Wound-healing assay The migratory ability of the MDA-MB-231 cells was measured using the in vitro wound-healing assay [56] . A monolayer of cells was grown to confluence in a six-well plate, and at experimental time zero, a scratch was made in each well using a pipette tip. The cells were washed twice with FBS-free medium before their subsequent incubation with culture medium in the absence (control) or presence of SP-141 at appropriate concentrations. In order to monitor the cell movement into the wounded area, five fields of each of the three wounds analysed per condition were photographed at 0, 4 and 20 h. Western blot analysis For the in vitro studies, cells were exposed to various concentrations of SP-141 for 24 h. In vivo tissue homogenates were prepared in RIPA buffer (100 mg tumour tissue per 1 ml RIPA) for the immunoblotting analysis. Cell lysates were fractionated with identical amounts of protein using SDS–PAGE and transferred to Bio-Rad trans-Blot nitrocellulose membranes (Bio-Rad Laboratories, Hercules, CA, USA) as described previously [54] , [55] , [56] . The nitrocellulose membrane was then incubated in blocking buffer (Tris-buffered saline containing 0.1% Tween 20 and 5% nonfat milk) for 1 h at room temperature. Then the membrane was incubated with the appropriate primary antibody overnight at 4 °C with gentle shaking. The membrane was washed three times with rinsing buffer (Tris-buffered saline containing 0.1% Tween 20) for 15 min, and then was incubated with goat anti-mouse/rabbit IgG-horseradish peroxidase-conjugated antibody (Bio-Rad) for 1 h at room temperature. After repeating the washes in triplicate, the protein of interest was detected using enhanced chemiluminescence reagents from PerkinElmer LAS Inc (Boston, MA, USA). Ubiquitination assay MCF-7 and MDA-MB-231 cells were co-transfected with MDM2 and ubiquitin plasmids, and were treated with SP-141 (0, 0.5 or 1 μM). Cell lysates were immunoprecipitated with corresponding antibodies, and the bound proteins were purified with protein G-Sepharose beads, resolved on SDS–PAGE and detected with an antiubiquitin antibody [56] . Immunofluorescence MCF-7 and MDA-MB-231 cells were seeded on coverslips in a 12-well plate at a density of 10,000 cells per well, allowed to attach overnight and treated with SP-141 (0 and 1 μM) for 24 h. The cells were fixed, and immunofluorescent staining was carried out as described previously [57] . Images were captured with a confocal microscope (Olympus America Inc, Center Valley, PA, USA). Mouse xenograft models of human cancer The animal protocol was approved by the Institutional Animal Use and Care Committee of Texas Tech University. Female athymic pathogen-free nude mice (nu/nu, 4–6 weeks) were purchased from Charles River Laboratories International Inc. (Wilmington, MA, USA). To establish MCF-7 human breast cancer xenografts [54] , [55] , [56] , each of the female nude mice was first implanted with a 60-day subcutaneous (s.c.) slow release oestrogen pellet (SE-121, 1.7 mg 17β-oestradiol/pellet; Innovative Research of America, Sarasota, FL, USA). Cultured MCF-7 cells were injected s.c. (5 × 10 6 cells, total volume 0.2 ml) into the left inguinal area of the mice on the following day. For the MDA-MB-468 xenograft model [54] , [55] , [56] , we used the same procedure as above, but without the oestrogen pellet. All animals were monitored for activity, physical condition, body weight and tumour growth. The tumour size was determined by caliper measurement in two perpendicular diameters of the implant every 3 days. The tumour weight (in g) was calculated using the formula: 1/2 a × b 2 , where ‘ a ’ is the long diameter and ‘ b ’ is the short diameter (in cm). The animals bearing human cancer xenografts were randomly divided into various treatment groups and a control group (10–15 mice per group). The untreated control group received the vehicle only. SP-141 was dissolved in PEG400:ethanol:saline (57.1:14.3:28.6, v/v/v) and was administered by i.p. injection at doses of 40 mg kg −1 per day, 5 days per week for 42 days (MCF-7 xenograft model) or 30 days (MDA-MB-468 xenograft model). At different time points of the experiments, xenograft tumours and other organs were removed, weighed and snap-frozen for western blot analysis, immunohistochemistry and haematoxylin and eosin (H&E) staining. In vivo assay for experimental cancer metastasis MDA-MB-231-Luc cells (1 × 10 6 , total volume 0.1 ml) were trypsinized and resuspended in serum-free medium and were intravenously injected into a tail vein of nu/nu mice [56] . These mice were then given a luciferase substrate (Caliper, Mountain View, CA, USA) and photographed using the IVIS Lumina XR in vivo imaging system (Caliper) on days 1, 8 and 15 to observe the in vivo cancer cell metastasis. The animals were treated by i.p. injection of SP-141 at 20 mg kg −1 per day, 5 days per week for 2 weeks. Same control group was used in another study [56] . H&E staining and immunohistochemistry The H&E staining was performed as described previously [58] . Briefly, freshly dissected tissues were fixed and embedded in paraffin. After being cut into 4-μm slices, the sections were deparaffinized and stained with Mayer’s Haematoxylin and Eosin solution. Finally, the sections were dehydrated and mounted with Permount in a fume hood. The results were analysed under a phase-contrast Olympus microscope (Olympus America Inc.). For the immunohistochemical staining, freshly dissected tissue was fixed in 10% neutral buffered formalin for 24–48 h. The tissue block was embedded in paraffin and cut to the desired thickness using a microtome, and was affixed on the slide. After several wash cycles, the tumour sections were blocked and incubated with an anti-human MDM2 antibody and pre-diluted streptavidin–peroxidase horseradish peroxidase conjugates using a staining kit (Dako North America Inc., CA, USA). The sections were counterstained with haematoxylin and were analysed under a phase-contrast Olympus microscope (Olympus America Inc) [58] . Statistical analysis Data were analysed using the Prism software version 6 (Graph Pad software Inc., San Diego, CA, USA). The Student’s t -test was used for comparisons between the two groups. The quantitative data are reported as means±s.e.m. from at least three independent experiments. Differences were considered statistically significant at P <0.05. All statistical tests were two-sided. How to cite this article: Wang, W. et al. The Pyrido[ b ]indole MDM2 inhibitor SP-141 exerts potent therapeutic effects in breast cancer models. Nat. Commun. 5:5086 doi: 10.1038/ncomms6086 (2014).